MinCD cell division proteins form alternating copolymeric cytomotive filaments During bacterial cell division, filaments of the tubulin-like protein FtsZ assemble at midcell to form the cytokinetic Z-ring. Its positioning is regulated by the oscillation of MinCDE proteins. MinC is activated by MinD through an unknown mechanism and prevents Z-ring assembly anywhere but midcell. Here, using X-ray crystallography, electron microscopy and in vivo analyses, we show that MinD activates MinC by forming a new class of alternating copolymeric filaments that show similarity to eukaryotic septin filaments. A non-polymerizing mutation in MinD causes aberrant cell division in Escherichia coli . MinCD copolymers bind to membrane, interact with FtsZ and are disassembled by MinE. Imaging a functional msfGFP-MinC fusion protein in MinE-deleted cells reveals filamentous structures. EM imaging of our reconstitution of the MinCD-FtsZ interaction on liposome surfaces reveals a plausible mechanism for regulation of FtsZ ring assembly by MinCD copolymers. In bacteria, precise positioning of the cytokinetic Z-ring at midcell is accomplished by a combination of two negatively regulating mechanisms, nucleoid occlusion and the Min system [1] , [2] , [3] . Nucleoid occlusion inhibits Z-ring assembly in the vicinity of the nucleoid [4] , [5] , whereas the Min system protects cell poles from abnormal division [2] . The E. coli Min system comprises proteins MinC, MinD and MinE. MinC, the FtsZ-interacting component of the system, is recruited to the membrane by MinD [6] , a deviant Walker A-type cytoskeletal ATPase (WACA) [7] . MinC and MinD together form the inhibitor complex that prevents Z-ring assembly anywhere but midcell [8] . In vitro studies revealed that MinD and all other WACAs form ATP sandwich dimers [9] , [10] , [11] , [12] . Dimerization leads to the exposure of a carboxy-terminal amphipathic helix (also called MTS, membrane-targeting sequence) that anchors MinD to the cytoplasmic membrane [13] . MinE stimulates MinD’s ATPase and dislodges the MinCD complex from the membrane [14] , [15] . The MinDE components of this system act as a Turing reaction–diffusion device [2] , [16] , leading to oscillation with MinC being the passenger. MinC is a dimeric two-domain protein whose amino-terminal domain (MinC N ) directly interacts with FtsZ and interferes with FtsZ’s ability to form the Z-ring [17] , [18] , but does not affect its GTPase activity or polymerization ability [19] . MinC’s C-terminal domain, MinC C , forms a constitutive dimer and interacts with MinD as well as with FtsZ [18] . Although at higher stoichiometric ratios MinC alters the rigidity of FtsZ polymers in vitro , MinC alone is not an efficient inhibitor in vivo [20] . This is probably because in cells FtsZ concentration is ~40-fold higher than that of MinC [21] , [22] . In vivo , MinD activates MinC by recruiting it to the membrane, forming an inhibitor complex that has much higher affinity for septal components [23] . Zhou and Lutkenhaus [24] isolated a mutation at the Switch II region of MinD that could recruit MinC to the septum but still failed to activate the latter. This suggested that MinC activation by MinD is more than just recruitment of MinC to the membrane. The mechanism of MinC activation by MinD, and how the MinCD inhibitor complex regulates Z-ring assembly, has so far remained unclear. Here, using in vitro and in vivo analyses, we show that MinC and MinD together form a new class of nucleotide-dependent, alternating copolymeric filaments. We present the near-atomic structure of the MinCD copolymers (first of a Walker A cytoskeletal ATPase family protein filament) and demonstrate that the MinCD copolymers interact with FtsZ filaments. Finally, our in vitro reconstitution of the MinCD-FtsZ complex on liposome membranes suggests a plausible mechanism for how substoichiometric levels of MinCD copolymers might regulate Z-ring assembly. Aquifex aeolicus MinC C –MinD co-crystal structure To understand the structural basis of MinC activation by MinD, we solved the MinC–MinD co-crystal structure. We used the C-terminal dimerization domain of A. aeolicus (Aa) AaMinC C with AaMinD, as MinC C has been reported to interact with MinD [18] . The AaMinC C –MinD (MinDΔ12D40A) co-crystal structure was solved at 2.7 Å resolution ( Fig. 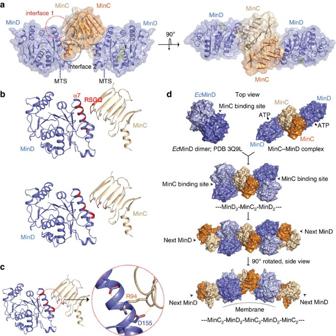Figure 1: MinCD co-crystal structure suggests a copolymeric filament. (a) Surface and cartoon representation of theA. aeolicusMinCD co-crystal structure showing an AaMinCCdimer (orange and wheat) sandwiched by two monomeric AaMinD(ΔC12, D40A) molecules (slate and light blue), bound to one ATP each. Two separate interfaces are highlighted with circles. Dotted blue lines show the position of the amphipathic helix (MTS) of MinD. (b) The MinC–MinD interface. Top: in red, residues that were previously identified as important for the MinC–MinD interaction12,20. Bottom: in red, residues that we found to make contacts in our AaMinCC-MinD co-crystal structure. (c) D155 of AaMinD helix7 (EcMinD D154) forms a tight salt bridge with R94 of MinC. Previously, both of these residues (seeSupplementary Fig. 1B) were identified as important for the MinC–MinD interaction18. (d) TheA. aeolicusMinCD co-crystal structure andE. coliMinD dimer structure (PDB 3Q9L) were used to build a composite filament model by sequential superimposition of MinDs from two crystal structures (seeSupplementary Movie 1). 1a , Table 1 and Supplementary Fig. 1E ). The MinCD co-crystals contained two molecules of MinC C and two molecules of MinD per asymmetric unit. The two MinC C β-helical domains engage in the same tight dimer as seen previously for Thermotoga maritima MinC C (PDB 1HF2) [17] . The AaMinC C dimer is sandwiched by two MinD molecules, each bound to ATP, but the MinDs did not form dimers in the crystal. Figure 1: MinCD co-crystal structure suggests a copolymeric filament. ( a ) Surface and cartoon representation of the A. aeolicus MinCD co-crystal structure showing an AaMinC C dimer (orange and wheat) sandwiched by two monomeric AaMinD(ΔC12, D40A) molecules (slate and light blue), bound to one ATP each. Two separate interfaces are highlighted with circles. Dotted blue lines show the position of the amphipathic helix (MTS) of MinD. ( b ) The MinC–MinD interface. Top: in red, residues that were previously identified as important for the MinC–MinD interaction [12] , [20] . Bottom: in red, residues that we found to make contacts in our AaMinC C -MinD co-crystal structure. ( c ) D155 of AaMinD helix7 (EcMinD D154) forms a tight salt bridge with R94 of MinC. Previously, both of these residues (see Supplementary Fig. 1B ) were identified as important for the MinC–MinD interaction [18] . ( d ) The A. aeolicus MinCD co-crystal structure and E. coli MinD dimer structure (PDB 3Q9L) were used to build a composite filament model by sequential superimposition of MinDs from two crystal structures (see Supplementary Movie 1 ). Full size image Table 1 Data collection and refinement statistics. Full size table The MinD-interacting sites on the MinC C dimer are located on opposite sides of the dimer, furthest away from the MinC C homodimer interface. Previous studies indicated that a highly conserved RSGQ motif within MinC C and helix 7 of MinD are critical for the MinCD interaction [12] , [20] ( Fig. 1b ). Satisfyingly, in our structure, the RSGQ motif (RAGQ in A. aeolicus ) of MinC and MinD helix 7 make up interface 1, one of two distinct interaction surfaces between the two molecules ( Fig. 1a,b and Supplementary Fig. 1A ). In interface 1, E162, D155 (from helix 7), D194, I195 and K197 (from helix 8) of MinD make significant contacts with R94, A95, D110, N112, K128 and R130 of the MinC C β-helix. In earlier studies, the highly conserved residues D155 (D154 in E. coli MinD) and R94 (RSGQ motif in E. coli MinC) were identified as important for MinC–MinD interaction ( Fig. 1c and Supplementary Fig. 1B ). The co-crystal structure also revealed a second interface between helix 8 of MinD and helix 3 (the C-terminal tail) from the other MinC C in the dimer ( Supplementary Fig. 1A ). However, helix 3, the C-terminal tail of MinC, is absent in many organisms. Previously, an E. coli MinD (EcMinD) dimer crystal structure had been solved (PDB 3Q9L). We combined our new crystal structure with the EcMinD dimer structure, revealing two interesting features ( Fig. 1d ). First, it is geometrically impossible to form a closed-symmetrical 2+2 dimer complex between MinC and MinD, given the MinC–MinD contacts we describe here. This is because MinD’s helix 7 is located close to the dimer interface on opposite ends of the MinD dimer and the RSGQ motifs on the MinC C dimer are located at opposite ends, furthest away from the dimer interface ( Supplementary Fig. 1D ). Second, to satisfy all the binding surfaces within and between the two dimer structures of MinC and MinD, translational symmetry is required: a filament in which a MinD dimer is followed by a MinC dimer, which is followed by a MinD dimer and so on. Using our knowledge of the MinC–MinC, MinD–MinD and MinC–MinD interactions, we then built a composite model of the MinCD filament ( Fig. 1d ). We used our new AaMinCD co-crystal structure (MinD-MinC 2 -MinD), the EcMinD dimer crystal structure (MinD 2 , PDB 3Q9L) and the safe assumption that AaMinD dimerizes in a similar manner to EcMinD. We first superimposed the EcMinD dimer structure (MinD 2 ) on each of the MinD molecules, at each side of the MinC dimer, in the MinD-MinC 2 -MinD structure, resulting in MinD 2 -MinC 2 -MinD 2 . We then superimposed another MinD-MinC 2 -MinD structure on the new MinDs at both ends, yielding MinD-MinC 2 -MinD 2 -MinC 2 -MinD 2 -MinC 2 -MinD. This process could be continued indefinitely and led to a curved copolymeric filament (~30° from one MinD dimer to another. Fig. 1d and Supplementary Movie 1 ). The membrane-binding surface of this filament, as indicated by the positions of the C-terminal amphipathic MinD helices (MTS), is at the concave side of the curved filament ( Fig. 1a,d ). MinC and MinD copolymerize to form an alternating copolymer To experimentally test filament formation, we used full-length, untagged E. coli MinC and MinD proteins in a light-scattering assay. EcMinD alone in the presence of ATP or ATP analogues did not show any increase in scattering ( Fig. 2a ). However, when ATP was added to a 1:1 mixture of MinC and MinD (the stoichiometry predicted from the structure, Fig. 1d ), we observed a dramatic increase in scattering intensity, indicative of formation of large-scale structures ( Fig. 2a ). Negative staining electron microscopy (EM) of the same sample showed large numbers of protein filaments ( Fig. 2c ). Consistent with our composite filament model in which filament formation requires only the C-terminal domain of MinC, E. coli MinC C also formed filaments with MinD ( Supplementary Fig. 1C ). To further confirm our results, we carried out similar experiments with untagged AaMinC and AaMinD proteins, and negative staining EM showed convincing protein filaments ( Fig. 2d ). During the course of these experiments, we found that the presence of tags at either terminus of MinD or at the C terminus of MinC greatly reduces the rate of filament formation ( Supplementary Fig. 2 ). 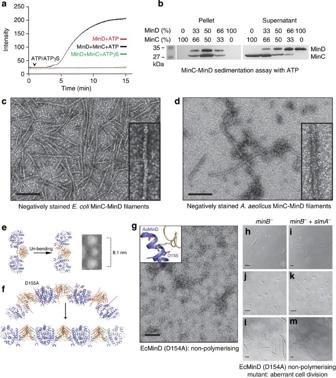Figure 2: MinC and MinD assemble into nucleotide-dependent copolymeric filaments. (a) Copolymerization of MinCD filaments as followed by 90° angle light scattering.E. coliMinD (15 μM) and MinC+MinD (each 15 μM) were incubated with ATP/ATPγS (1 mM) at 25 °C.In vitrocritical concentration for MinCD filament formation was determined to be ~7 μM of each protein. (b)A. aeolicusMinC and MinD were mixed in different ratios in a co-sedimentation assay with ATP. Left: maximum pelleting occurs at a molar ratio of 1:1 (SDS–PAGE).E. coli(c) andA. aeolicus(d) MinCD copolymeric filaments observed by negative staining EM. Scale bar, 100 nm. (e) The MinCD co-crystal structure is intrinsically bent (see alsoFig. 1a,d). Right: the structure after manual unbending by rotating a flexible loop within MinCC(Supplementary Fig. 3G). A low-pass filtered building block of a MinCD copolymer correlates well with the MinCD co-crystal structure and has a similar repeat distance. (f) Composite model of the straightened MinCD filament. (g) A non-polymerizing mutant: EcMinD (D154A) at the MinC–MinD interface disrupts filaments (D155 in AaMinD). (h–m)E. coli minB−andminB−slmA−mutants were transformed with low-copy plasmid pJB210 containing theminBoperon. Bright-field micrographs ofminB−andminB−slmA−mutants showing non-complemented cells (h,i), or complemented with pJB210 plasmid (j,k). MinCD non-polymerizing mutant (D154A) fails to complement both phenotypes (l,m). Scale bars, 5 μm. Figure 2: MinC and MinD assemble into nucleotide-dependent copolymeric filaments. ( a ) Copolymerization of MinCD filaments as followed by 90° angle light scattering. E. coli MinD (15 μM) and MinC+MinD (each 15 μM) were incubated with ATP/ATPγS (1 mM) at 25 °C. In vitro critical concentration for MinCD filament formation was determined to be ~7 μM of each protein. ( b ) A. aeolicus MinC and MinD were mixed in different ratios in a co-sedimentation assay with ATP. Left: maximum pelleting occurs at a molar ratio of 1:1 (SDS–PAGE). E. coli ( c ) and A. aeolicus ( d ) MinCD copolymeric filaments observed by negative staining EM. Scale bar, 100 nm. ( e ) The MinCD co-crystal structure is intrinsically bent (see also Fig. 1a,d ). Right: the structure after manual unbending by rotating a flexible loop within MinC C ( Supplementary Fig. 3G ). A low-pass filtered building block of a MinCD copolymer correlates well with the MinCD co-crystal structure and has a similar repeat distance. ( f ) Composite model of the straightened MinCD filament. ( g ) A non-polymerizing mutant: EcMinD (D154A) at the MinC–MinD interface disrupts filaments (D155 in AaMinD). ( h – m ) E. coli minB − and minB − slmA − mutants were transformed with low-copy plasmid pJB210 containing the minB operon. Bright-field micrographs of minB − and minB − slmA − mutants showing non-complemented cells ( h , i ), or complemented with pJB210 plasmid ( j , k ). MinCD non-polymerizing mutant (D154A) fails to complement both phenotypes ( l , m ). Scale bars, 5 μm. Full size image We then carried out a co-sedimentation assay with simultaneously increasing and decreasing amounts of untagged AaMinD and AaMinC, respectively, in the presence of ATP ( Fig. 2b ). AaMinC or AaMinD alone did not sediment when incubated with ATP and maximum pellet formation was observed at a molar ratio of 1:1. We concluded that MinC and MinD form copolymeric protein filaments with a stoichiometric ratio of 1:1. More detailed analysis of negative stain EM images of EcMinCD filaments revealed different views. The most easily interpretable view showed pairs of flat and straight filaments ( Supplementary Fig. 3A–D ). Careful inspection suggested the individual filaments were staggered relative to each other. Low-resolution filtering of small segments of these filaments revealed that they are made of arrowhead-shaped building blocks that matched very well the shape of the MinCD complex in our crystal structure ( Fig. 2e ). A Fourier transform of the MinCD filaments revealed an axial repeat of ~7.8 nm, which is consistent with the equivalent distance (8.1 nm) in the MinCD co-crystal structure ( Supplementary Fig. 3B,E ). In our composite filament model, the MinCD filament is curved ( Figs 1d and 2f , and Supplementary Fig. 3E ). However, we found it can be unbent easily by rotating a C-terminal loop of MinC C , without any change at the MinC–MinD interface ( Supplementary Fig. 3E,G ). This leads to a filament that is completely straight, as one would expect, as MinCD binds to almost flat membranes in cells when cellular dimensions are considered. We compared a staggered pair of our straightened composite filament model with the appearance of MinCD filaments in EM and they correlate well ( Supplementary Fig. 3F,C,D ). Other views of MinCD filaments seen by EM ( Fig. 2c ) can be interpreted as small twisted bundles of the basic staggered pair. We concluded that EM analysis supports the notion that MinCD form the alternating copolymeric filaments depicted in Fig. 1d . We then mutated a key residue within the MinC–MinD interface, EcMinD(D154A), and mutating this residue was expected to interfere with the MinC–MinD interaction, which we now show leads to filaments ( Fig. 1c ). The D154A mutation completely abolished MinCD filament formation in vitro ( Fig. 2g ). We tested this non-polymerizing mutant in a complementation assay (see Supplementary Note 1 ) to rescue minB- and minB- slmA- phenotypes in E. coli ( Fig. 2h,i ). Unmodified minB operon provided in an appropriate plasmid did complement ( Fig. 2j,k ); however, the non-polymerizing mutant introduced into the minB operon did not ( Fig. 2l,m ), suggesting the contact between MinC and MinD dimers that causes copolymerization is important for biological function. However, as the interface between MinC and MinD at the same time causes copolymerization and also recruits MinC to MinD (and to the membrane), it is principally not possible to disentangle these functions. This is because binding of MinC to MinD will inevitably lead to filaments because of the two proteins being dimers and the position of their interaction surfaces ( Supplementary Fig. 1D ). MinCD filaments form a new class of cytomotive filaments The MinCD copolymeric filaments remained unchanged for hours as observed by subsequent negative staining EM (not shown). Previous studies showed that MinE displaced MinC from the membrane-bound MinCD complex and stimulated the ATPase activity of MinD, leading to the disruption of MinD dimers. To test the effect of MinE on MinCD filaments, we added MinE to the same experiment as described in Fig. 2a . Scattering dropped almost to the baseline, suggesting disruption of the filaments ( Fig. 3d ). EM images of the same sample confirmed that the filaments had indeed completely disappeared ( Supplementary Fig. 4B ). This confirmed that MinE disrupts MinCD filaments and suggested that the MinCD filaments are regulated by intrinsic nucleotide turnover, making them belong to the class of cytomotive cytoskeletal filaments, with actin and tubulin being the most prominent members [25] . 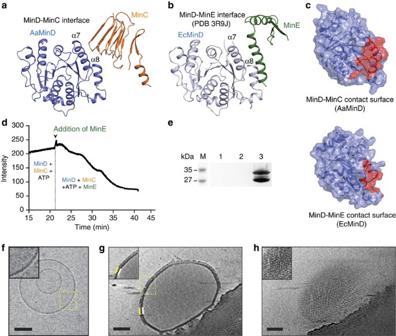Figure 3: MinCD filaments bind to membrane and are disassembled by MinE. (a,b) In the AaMinCD complex and EcMinDE complex (PDB 3R9J), MinC and MinE compete for a very similar binding surface on MinD. (c) Surfaces of AaMinD and EcMinD showing their MinC and MinE interaction interfaces (red). (d) EcMinCD filament disassembly on addition of MinE. (e) Low-speed sedimentation assay showing binding of EcMinCD filaments to liposomes. SDS–PAGE of pellets only, lanes: 1, liposomes; 2, MinCD filaments; 3, liposomes and MinCD filaments. (f–h) ECT of MinCD filament-decorated liposomes. Insets were low-pass filtered. (f) Liposomes without protein. (g) Additional layer on the membrane surface (white) caused by addition of MinCD (yellow). (h) Surface of the liposome showed a MinCD filament network. Scale bar, 100 nm. Figure 3: MinCD filaments bind to membrane and are disassembled by MinE. ( a , b ) In the AaMinCD complex and EcMinDE complex (PDB 3R9J), MinC and MinE compete for a very similar binding surface on MinD. ( c ) Surfaces of AaMinD and EcMinD showing their MinC and MinE interaction interfaces (red). ( d ) EcMinCD filament disassembly on addition of MinE. ( e ) Low-speed sedimentation assay showing binding of EcMinCD filaments to liposomes. SDS–PAGE of pellets only, lanes: 1, liposomes; 2, MinCD filaments; 3, liposomes and MinCD filaments. ( f – h ) ECT of MinCD filament-decorated liposomes. Insets were low-pass filtered. ( f ) Liposomes without protein. ( g ) Additional layer on the membrane surface (white) caused by addition of MinCD (yellow). ( h ) Surface of the liposome showed a MinCD filament network. Scale bar, 100 nm. Full size image Comparison between a previously published MinD–MinE co-crystal structure (PDB 3R9J) [26] and our MinD–MinC complex structure provided an additional explanation for the mechanism of MinCD filament disruption, apart from the expected ATPase activation of MinD by MinE that leads to MinD dimer disassembly ( Fig. 3a,b ). Superposition revealed that the MinE contact helix competes with MinC for binding to MinD and the interface surfaces clearly overlap ( Fig. 3c and Supplementary Fig. 4A ), as was indicated previously [6] , [15] . MinCD copolymers bind to lipid membranes The active state of the MinCD inhibitor complex is bound to the membrane in cells. To examine whether the MinCD copolymeric filaments would bind to membrane, we used a low-speed liposome sedimentation assay ( Fig. 3e ). MinCD filaments did not sediment on their own at this low-centrifugal force, but when MinCD filaments were added to the liposomes they co-sedimented. This suggested that MinCD filaments bind to liposomes. To visualize the arrangement of the MinCD filaments on the liposome surface, we used electron cryotomography (ECT). Addition of MinCD filaments distorted most of the liposomes ( Fig. 3f,g ), although none were transformed into narrow tubes as caused by MinD or MinD’s amphipathic helix alone ( Supplementary Fig. 5 ). With MinCD, we could see very prominent structures decorating the surfaces of the liposomes ( Fig. 3g,h and Supplementary Movie 2 ). Sections through the ECT reconstructions of decorated liposomes revealed that the MinCD copolymers formed filamentous networks on the liposome surface with an axial spacing of ~8 nm, very similar to that observed in MinCD filaments in negative stain ( Supplementary Fig. 3B ). We concluded that MinCD filaments bind and decorate membranes. Biological function of MinCD copolymers The MinDE component of the MinCDE system acts as the Turing reaction–diffusion device that transports MinC, whereas the MinCD component forms an active inhibitor complex that prevents Z-ring assembly. As MinD is involved in both functions, we examined putative, non-essential roles of MinCD copolymers in Min oscillation (as it had previously been shown that MinDE oscillation occurs without MinC [2] , [27] ) as well as possible roles in the FtsZ inhibition process. Our in vivo complementation assay demonstrated that MinCD copolymers seem not to interfere with Min oscillation, as non-polymerizing green fluorescent protein (GFP) fusions of MinC or MinD still oscillate ( Supplementary Fig. 6 and Supplementary Table 2 ). While performing these experiments, it became apparent that most of the MinC or MinD GFP fusion proteins were non-functional in our complementation assay. To exclude the possibility that non-functional proteins hide specific effects, new msfGFP-MinC fusion proteins were generated that were fully functional in cell division inhibition, supported oscillation and polymerized into MinCD filaments ( Supplementary Note 1 and Supplementary Figs 6 and 7 ), leading to the same conclusion that MinC probably has no or only very limited influence on oscillation of MinDE. Thus, we next examined the role of MinCD copolymers in regulating FtsZ-based cell division. For this, we first added pre-formed MinCD copolymeric filaments and GMPCPP-polymerized FtsZ filaments to liposomes and imaged them with ECT ( Fig. 4a,c and Supplementary Movie 3 ). Sections through ECT reconstructions of liposomes clearly showed two additional layers on top of the bilayer ( Fig. 4a,c ). Control experiments with only liposomes showed just bilayers, whereas experiments with liposomes and MinCD copolymers showed one additional layer decorating the liposome surface, as already shown ( Figs 4a and 3g ). The surface view of the tomographic reconstruction revealed FtsZ filaments covering up the characteristic beady appearance of MinCD filaments ( Fig. 4d in contrast to Fig. 3h ). A Fourier transform of the layer immediately next to the bilayer showed an axial repeat distance of ~8 nm, which is consistent with the repeat distance of MinCD copolymeric filaments of ~7.8 nm ( Fig. 4e and Supplementary Fig. 3B ). Fourier transform of the second layer, further away from the bilayer, showed a repeat distance of ~4 nm, which corresponds to the FtsZ axial repeat distance ( Fig. 4e ) [28] . In our ECT data, the distance measured from the liposome membrane, over MinCD to the FtsZ polymers, is ~16 nm, which is consistent with the measured in vivo distance in cellular ECT data of Caulobacter crescentus cells [29] . 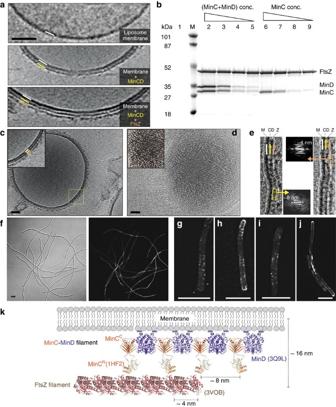Figure 4: MinCD copolymers recruit FtsZ filaments onto liposome surfaces. (a) ECT of EcMinCD and EcFtsZ filament decorated liposomes. Top: liposome only; middle: MinCD added, additional layer appeared (yellow); bottom: MinCD and FtsZ added, two additional layers (yellow and orange). (b) Sedimentation assay of EcFtsZ filaments with EcMinC alone (right) or EcMinCD (left). Varying amounts of MinC (4.5, 2.25, 0.9 and 0.45 μM, lanes 6–9) or MinCD (4.5, 2.25, 0.9 and 0.45 μM each, lanes 2–5) were added to 4.5 μM of FtsZ. Lane 1: MinCD did not co-sediment at 4.5 μM each, as below critical concentration for MinCD filament formation without lipid. (c) Vesicle double-coated with MinCD and FtsZ filaments (ECT section). (d) The surface view was different fromFig. 3h, because it was now covered with FtsZ filaments (ECT surface view). (e) Fourier transforms of the two layers on the liposomes confirmed that the layer next to the membrane consisted of MinCD copolymers (axial repeat ~8 nm) and the other contained FtsZ filaments (axial repeat ~4 nm). Scale bar, 50 nm. (f) Representative bright-field and fluorescent micrographs ofminB−mutant, complemented with a pJB210-derived plasmid (pDG62) containing a fully functional msfGFP-MinC fusion (N-terminal msfGFP), but lacking MinE (confocal microscopy). Cells at mid-log phase show a strong filamentous phenotype, presumably MinCD now inhibits cell division everywhere in the cell. (g–j) Super-resolution imaging of these cells (SIM) showed distinct filamentous/ring-like structures associated with the membrane presumably in the form of MinCD filaments, as they were not disassembled by MinE. Scale bar, 5 μm. (k) Model of how MinCD and FtsZ filaments arrange on the membrane. The MinCD alternating copolymer filament binds to the membrane through MinD.T. maritimaMinC (PDB 1HF2) was superimposed on the MinCD co-crystal structure to generate a model including N-terminal MinC domains. FtsZ protofilament is fromStaphylococcus aureus(PDB 3VO8). MinCD bridges the distance from the membrane to the FtsZ filaments in the Z-ring and the two filament systems form copolymers. We propose that the MinCD filaments select FtsZ filaments over monomers through avidity and inhibit lateral interactions of the FtsZ filaments with each other. Inhibition of lateral interactions might involve blocking of lateral FtsZ–FtsZ binding sites, or may be subtle, through rotation of the FtsZ protofilaments along their long axis. Figure 4: MinCD copolymers recruit FtsZ filaments onto liposome surfaces. ( a ) ECT of EcMinCD and EcFtsZ filament decorated liposomes. Top: liposome only; middle: MinCD added, additional layer appeared (yellow); bottom: MinCD and FtsZ added, two additional layers (yellow and orange). ( b ) Sedimentation assay of EcFtsZ filaments with EcMinC alone (right) or EcMinCD (left). Varying amounts of MinC (4.5, 2.25, 0.9 and 0.45 μM, lanes 6–9) or MinCD (4.5, 2.25, 0.9 and 0.45 μM each, lanes 2–5) were added to 4.5 μM of FtsZ. Lane 1: MinCD did not co-sediment at 4.5 μM each, as below critical concentration for MinCD filament formation without lipid. ( c ) Vesicle double-coated with MinCD and FtsZ filaments (ECT section). ( d ) The surface view was different from Fig. 3h , because it was now covered with FtsZ filaments (ECT surface view). ( e ) Fourier transforms of the two layers on the liposomes confirmed that the layer next to the membrane consisted of MinCD copolymers (axial repeat ~8 nm) and the other contained FtsZ filaments (axial repeat ~4 nm). Scale bar, 50 nm. ( f ) Representative bright-field and fluorescent micrographs of minB − mutant, complemented with a pJB210-derived plasmid (pDG62) containing a fully functional msfGFP-MinC fusion (N-terminal msfGFP), but lacking MinE (confocal microscopy). Cells at mid-log phase show a strong filamentous phenotype, presumably MinCD now inhibits cell division everywhere in the cell. ( g – j ) Super-resolution imaging of these cells (SIM) showed distinct filamentous/ring-like structures associated with the membrane presumably in the form of MinCD filaments, as they were not disassembled by MinE. Scale bar, 5 μm. ( k ) Model of how MinCD and FtsZ filaments arrange on the membrane. The MinCD alternating copolymer filament binds to the membrane through MinD. T. maritima MinC (PDB 1HF2) was superimposed on the MinCD co-crystal structure to generate a model including N-terminal MinC domains. FtsZ protofilament is from Staphylococcus aureus (PDB 3VO8). MinCD bridges the distance from the membrane to the FtsZ filaments in the Z-ring and the two filament systems form copolymers. We propose that the MinCD filaments select FtsZ filaments over monomers through avidity and inhibit lateral interactions of the FtsZ filaments with each other. Inhibition of lateral interactions might involve blocking of lateral FtsZ–FtsZ binding sites, or may be subtle, through rotation of the FtsZ protofilaments along their long axis. Full size image To further confirm that untagged, full-length MinCD proteins do not depolymerize FtsZ as indicated by the liposome imaging ( Fig. 4a ), we performed a pelleting assay based on FtsZ, this time below the critical concentration so that MinCD is not expected to form filaments ( Fig. 4b ). We did not observe any difference in FtsZ pelleting either with MinC alone or with MinC and MinD. However, MinC alone co-sedimented with FtsZ polymers and co-sedimentation increased with MinC concentration. Furthermore, we found a roughly two-fold increase in MinC co-sedimentation in the presence of MinD compared with MinC alone. This was true for GTP- and GMPCPP-polymerized FtsZ filaments. These data suggested the following: first, MinC alone or MinCD together do not affect the polymerization of FtsZ subunits into filaments or their disassembly; second, MinC binding to FtsZ is specific; and finally, MinD increases the cooperativity of MinC binding to FtsZ polymers. If MinD increases the cooperativity of MinC binding on the FtsZ polymers through filament formation as described here, this would mean that MinCD copolymers are more effective in antagonizing FtsZ filaments than MinC alone, given that the critical concentration for MinCD filament formation is lowered when polymerizing on FtsZ filaments and/or membrane ( Supplementary Fig. 8 ). This raises the enticing possibility that membrane-bound MinCD filaments might bind specifically to FtsZ filaments over monomers to regulate Z-ring assembly. Together these analyses confirmed that membrane-bound MinCD copolymers do not disrupt FtsZ filaments, instead MinCD filaments poise MinC for binding to FtsZ filaments, which are at quite some distance from the membrane. In vivo imaging of MinCD copolymers Finally, we imaged MinCD filaments in live E. coli cells. We used the minB − strain and introduced the minB operon with a low copy number plasmid (pDG57) containing our fully functional N-terminal msfGFP-MinC fusion. Initial attempts to image MinCD filaments failed, presumably due to rapid oscillation of the Min proteins. Therefore, we deleted MinE from the plasmid, as this should stop Min oscillation and will also stabilize the MinCD filaments. Introduction of a MinE-deleted plasmid (pDG62), containing a functional msfGFP-MinC, to the minB − strain, resulted in long filamentous cells, as cell division is inhibited everywhere as observed in earlier studies ( Fig. 4f ) [30] . However, contrary to the previous interpretation, deletion of MinE did not result in a homogeneous distribution of Min proteins [31] , as confocal micrographs showed a very inhomogeneous distribution of fluorescence in the cytoplasm and on the membrane ( Fig. 4f ). Structured illumination microscopy (SIM) showed the presence of distinct elongated polymers on the membrane and also ring-like structures ( Fig. 4g–j ), presumably in the form of MinCD copolymers. Thus, we confirmed that MinCD filaments exist in E. coli and are made dynamic by MinE. In this study, we have discovered that the bacterial cell division proteins MinC and MinD together form a new class of alternating copolymeric cytomotive filaments, and suggest that the membrane-bound MinCD copolymers constitute the active inhibitor complex that spatially regulates Z-ring assembly. MinD belongs to the WACA family of widely conserved bacterial proteins that play critical roles in diverse cellular processes [25] , [32] , [33] , [34] . Some previous studies have indicated that WACA proteins themselves, including MinD, assemble into ATP-dependent filaments, while others failed to observe higher-order assemblies [35] , [36] , [37] , [38] , [39] . We also did not observe any filaments and provide explanations for the opposing findings in the literature. Although it is difficult to be sure, we believe two artefacts common in negative staining EM might have been previously mistaken for WACA filaments: uranyl acetate needle-like crystals and contaminating cellulose fibres ( Supplementary Note 2 , compare Supplementary Figs 9 and 10 ). However, MinD readily formed nucleotide-dependent, cytomotive copolymeric filaments in the presence of MinC. Using X-ray crystallography, EM and biochemical methods, we have described the structure of the MinCD copolymers and provided an atomic model. In vitro , and without membrane or FtsZ filaments, the critical concentration for MinCD filament formation was estimated to be ~ 7 μM (based on the disappearance of filaments after subsequent negative staining EM). Cellular concentrations of MinC and MinD are lower and were previously estimated to be around ~ 0.7 μM for MinC and ~5 μM for MinD [22] , [40] . However, in vivo polymerization will be facilitated by cooperative assembly on the membrane, as reported, for example, for septins and dynamins [41] , [42] . We tested this by adding MinCD proteins to liposomes at much lower concentrations than the estimated critical concentration for MinCD filament formation in solution. Indeed, we could detect decoration of liposomes by MinCD filaments at concentrations as low as 0.5 μM ( Supplementary Fig. 8 ). In addition, considering cellular crowding and the presence of FtsZ filaments, which provide another surface for cooperative assembly, this suggests that MinCD filaments do form in E. coli cells. Imaging the MinCD filaments in a MinE deletion strain, where they should be stable, supported the idea that MinCD filaments occur in vivo. Unfortunately, it is currently not possible to reliably image at endogenous levels of MinC with SIM. Hence, we had to use a low-copy number plasmid ( n ~5), pJB210, carrying the entire minB operon, including natural promoters. pJB210 has been used previously to complement min- phenotype [30] , [43] and it complements the min- and min- slmA- phenotypes very well in our complementation assays ( Fig. 2j,k ). Currently, it is not obvious to us whether the finding of MinCD co-filaments would be transferrable to other WACA systems, most notably the DNA segregation systems of the ParAB type. ParB is thought to be the MinE equivalent of these systems, as it activates the ATPase in ParA, while DNA acts as the matrix (surface) instead of the membrane [44] . It is interesting to note that ParBs contain a constitutive dimerization domain [45] , which makes us speculate that ParB may contain both functions of MinC and MinE in one protein, possibly switched by the presence or absence of DNA. The MinCD filaments differ from actin-like and tubulin-like cytomotive filaments in two major ways. First, MinCD filaments consist of two structurally unrelated proteins that form a filament consisting of alternating dimers with two-fold axes, making the resulting filaments non-polar, somewhat reminiscent of septin filaments, with which MinD shares strong structural similarity [25] , [46] . Given this similarity, the MinC C-terminal β-helical domains would then be functionally equivalent to the septin N- and C-terminal extensions (NC-dimer interfaces) [46] that facilitate the septin G–domain dimer interactions, which enable filaments. Furthermore, septins polymerize along microtubules [47] and we show here that MinCD filaments bind to filaments of FtsZ, the bacterial tubulin homologue. Second, the ATPase activity is stimulated by an external protein, MinE, which moves independently, leading to the possibility of pattern formation. In contrast, nucleotide hydrolysis is self-activated on polymerization in all actin-like and tubulin-like proteins. Previous in vivo studies suggested that MinD augments MinC’s inhibitory activity about 25-to 50-fold by forming an active inhibitor complex [23] . We suggest here that the membrane-bound MinCD copolymers constitute the active inhibitor complex that spatially regulates Z-ring assembly. In our new model ( Fig. 4k and Supplementary Fig. 11 ), membrane-bound MinCD copolymers bind to membrane and FtsZ filaments with higher affinity over FtsZ monomers because of cooperativity (avidity effect) and may alter their structural integrity. Or, MinCD filaments could rotate FtsZ protofilaments around their longitudinal axis, such that lateral interactions between FtsZ filaments are no longer supported, thus sub-stoichiometrically impeding Z-ring function. This new model of FtsZ inhibition might explain how ~ 40 times fewer MinC molecules than FtsZ interfere with FtsZ’s function [21] , [22] . Independent of MinCD filaments, using the excess of MinD over MinC in cells, continuous oscillation of the Min system is essential for differential localization of all three components along the length of the cell. In this context, it is worth mentioning that MinE has been reported to form a ring-like structure predominantly at midcell [48] , and this could explain why Z-ring formation is limited in such a small band, as MinE will take apart MinCD filaments, which we have now identified as the active Z-ring inhibitor complex. Expression vectors For EM and light-scattering experiments, full-length MinD from E. coli , A. aeolicus , Bacillus subtilis , T. maritima , Archaeoglobus fulgidus ; full-length MinC from E. coli , A. aeolicus ; and full-length MinE from E. coli were amplified from genomic DNA (ATCC) and cloned between the NdeI and SapI sites of vector pTYB1/pTXB1 (New England Biolabs, Amp R ). This produced expression plasmids of a C-terminal, cleavable (intein+chitin binding domain) tag. Importantly, subsequent removal of the tag left no extra residues at either end of the protein. For crystallization trials, MinC C (aa 82–201), MinC and MinD were amplified from A. aeolicus genomic DNA and cloned between the NdeI and BamHI sites of vector pHis17 (ref. 49 ). This added eight extra residues, GSHHHHHH at the C terminus of the desired protein. The MinD construct used for MinC–MinD complex crystallization included the mutation D40A to reduce the rate of ATP hydrolysis and was truncated by 12 amino acids at the C terminus (ΔX12) to increase solubility, by removing the amphipathic helix (MTS). The monomeric MinD structure was solved from a similar MinD(ΔX13) construct Ec FtsZ was cloned in the pET28a vector (Kan R ) without any tag. GFP- or mCherry-tagged MinC and MinD, for purification purpose, were always cloned in pTXB1 vector between the NdeI and SapI sites. Protein expression and purification For all constructs, C41 cells were transformed and grown in 2 × TY media at 37 °C. Expression was induced at OD 600 nm 0.6 by adding IPTG (isopropyl-β- D -thiogalactoside) to a final concentration of 1 mM. After induction, cells were grown at 20°C for 20 h, harvested by centrifugation at 4,000 g and snap frozen in liquid nitrogen. For pTYB1-MinD constructs ( Supplementary Table 1 ), cells were re-suspended in 25 mM Tris-Cl, 1 mM NaN 3 and 1 mM EDTA, pH 8 (buffer A), and lysed in a cell disruptor at 25 kPSI at 4 °C (Constant Systems). Lysate was cleared by centrifugation at 20,000 g and the supernatant was loaded on a chitin affinity column. The protein was cleaved on the column by incubating with 50 mM dithiothreitol overnight at 4 °C and the eluted protein was then further purified by ion exchange chromatography (GE Healthcare HiTrap Q HP, 25 mM Tris-Cl, 100–500 mM NaCl gradient, pH 8) and finally by size-exclusion chromatography (GE Healthcare HiPrep 26/60 Sephacryl S200, 25 mM Tris-Cl, 1 mM NaN 3 , pH 8). pTYB1/pTXB1-MinC, -MinC C and -MinE constructs ( Supplementary Table 1 ) were also purified in a very similar way, except the cell pellets were dissolved in buffer B (buffer A plus 150 mM KCl) and the final size exclusion was also carried out in buffer B. mCherry- or GFP-tagged MinC and MinD proteins were purified in a similar way as untagged MinC and MinD proteins. For pHis17-MinD and -MinC constructs (with a C-terminal hexa-histidine tag), cells were dissolved in 25 mM Tris-Cl, 300 mM NaCl, 1 mM NaN 3 and 1 mM EDTA, pH 7, the supernatant was extracted as described above, passed through a nickel column (HisTrap, GE Healthcare) and eluted with a 0–1 M imidazole gradient. Eluted protein was further purified by size-exclusion chromatography (GE Healthcare HiPrep 26/60 Sephacryl S200, 25 mM Tris-Cl, 300 mM NaCl and 1 mM NaN 3 , pH 7). EcFtsZ was purified by ammonium sulfate precipitation, followed by ion exchange and finally size-exclusion chromatography in buffer A but pH 7. The sizes of all proteins were first estimated by SDS–PAGE and confirmed by electrospray ionization mass spectrometry. Crystallization A. aeolicus MinC C -MinD(ΔC12), D(40)A co-crystals were generated using the LMB’s high-throughput crystallization facility [50] and grown at 4 °C using the sitting-drop vapour diffusion method in MRC crystallization plates mixing 100 nl of protein solution with 100 nl reservoir solution containing 35 % PEG 200, 0.25 M CHES, pH 9.5. Crystals were cryoprotected in reservoir solution and flash frozen in liquid nitrogen. A. aeolicus MinD(ΔC13) crystals were grown using a similar method but at room temperature with a solution containing 18 % PEG 2000 MME, 200 mM MgCl 2 , 100 mM NaOAc, pH 5.0. In this case, crystals were cryoprotected in 20 % PEG 2000 MME, 40% PEG 400, 250 mM MgCl 2 and flash frozen in liquid nitrogen. Structure determination Diffraction images were collected at European Synchrotron Research Facility (ESRF, Grenoble, France) beamlines id23eh1 and id23eh2. Data were processed with XDS and SCALA [51] , [52] , [53] , and phases were calculated by molecular replacement using PHASER [54] . We used A. fulgidus MinD-like protein (PDB 1HYQ) [55] to obtain phase information for Aquifex MinD(ΔC13) and finally Aquifex MinD(ΔC13) was used to phase the MinC C -MinD (ΔC12), D(40)A complex data set to 2.7 Å. Models were built manually with MAIN [56] and refined with PHENIX [57] . X-ray data and refinement statistics are given in Table 1 . Light-scattering assay Full-length, untagged E. coli proteins (at 15 μM concentration) were used for this assay. Before the experiment, individual proteins were spun at 250,000 g in a Beckman TLA 100 rotor to remove aggregates. Assembly and disassembly of MinCD filaments were monitored in a 90° angle light-scattering spectrophotometer (Varian Cary Eclipse) with both the excitation and emission wavelengths set at 400 nm. Co-pelleting assay For the MinCD co-pelleting assay, full-length, untagged A. aeolicus proteins were used. Before the experiment, individual proteins were pre-spun at 250,000 g in a Beckman TLA 100 rotor to remove aggregates and protein concentrations were adjusted to 50 μM as stock solution. MinC and MinD proteins were mixed in reaction buffer (25 mM Tris-Cl, 1 mM NaN 3 and 100 mM KCl, pH 7.5) in different ratios, and ATP and MgCl 2 were added to a final concentration of 1 mM. At 100%, individual protein concentrations were 24 μM. The reaction mix was incubated at 25 °C for 15 min, spun at 250,000 g for 20 min and the supernatant and pellets were analysed by SDS–PAGE. For the MinCD-FtsZ co-pelleting assay, everything was similar but proteins used were from E. coli , reaction buffer pH 7.0 and the highest protein concentrations used was 4.5 μM. Liposome co-sedimentation assay Liposomes were prepared using E. coli total lipid extract (Avanti Polar Lipids) in reaction buffer (25 mM Tris-Cl, 1 mM NaN 3 and 100 mM KCl, pH 7.0) and mixed with preformed MinCD filaments. The reaction mix was incubated at 25 °C for 15 min. After the specified times, liposomes were sedimented by using a tabletop centrifuge at 16,000 g centrifugal force for 20 min. Negative stain EM Full-length, untagged MinC and MinD proteins were mixed to an individual final concentration of 15 μM in reaction buffer (25 mM Tris-Cl, 1 mM NaN 3 and 100 mM KCl, pH 7.5) and polymerization was initiated by addition of 1 mM ATP and 1 mM MgCl 2 . The reaction mix was then incubated at 25 °C for 15 min, applied onto a carbon-coated EM grid and stained with 1 % (wt/vol) uranyl acetate. Images were recorded using a Tecnai 12 electron microscope (FEI) at 120 kV and a charge-coupled device camera. Electron cryomicroscopy and tomography Specimens were plunge-frozen onto a Quantifoil R2/2, Cu/Rh holey carbon grid using an FEI Vitrobot (FEI Company, USA) and imaged with an FEI Tecnai G2 Polara electron microscope operating at 300 kV and equipped with a Gatan energy filter and 4 × 4 k Gatan Ultrascan charge-coupled device camera (binned to 2 × 2 k). For tomography, samples were imaged using a FEI Titan Krios TEM operating at 300 kV, equipped with a 4 k × 4 k K2 Summit direct electron detector at a magnification of 26 k, corresponding to a pixel size of 0.45 nm (for K2) at the specimen level. Tilt series were acquired using SerialEM software [58] between ±55° with 1° increment. The defocus was set between 5 and 8 μm, and the total dose for each tilt series was around 120 e Å −2 . Tilt series was aligned using the fiducial markers and IMOD software package and reconstruction was computed using simultaneous iterative reconstruction technique [59] , [60] . Plasmids, strains, growth media, and microscopy A detailed list of all the plasmids used in this study are given in Supplementary Table 1 . All strains used for the complementation assay are derivatives of MG1655. E. coli minB − (ΔlacIZYA::frt ΔminCDE::frt) and minB − slmA − (ΔlacIZYA::frt ΔminCDE::frt ΔslmA::frt) mutants were transformed with the appropriate plasmids. A single colony was inoculated into minimal M9 media supplemented with 0.2% casamino acids, 0.2% maltose and spectinomycin (100 μM) and grown overnight. The culture was then diluted 1:100 in LB media containing spectinomycin (100 μM) and grown until mid-log phase (OD 600 nm 0.5). Cells were taken from the growth media, mounted onto an agarose pad and visualized by either confocal or SIM. Confocal microscopy was performed using a Zeiss LSM780 confocal microscope, equipped with a × 63 oil immersion objective lens. For super-resolution microscopy, mid-log phase cells were added onto an agarose pad, covered with Zeiss high-performance coverslip and imaged using a Zeiss Elyra super-resolution SIM system equipped with a Zeiss × 63 oil immersion objective lens. Construction of chromosomal msfGFP fusion The min operon encoding monomeric superfolder GFP (msfGFP) sandwich fusion to MinC was PCR amplified from plasmid pDG61 ( Supplementary Table 1 ) and cloned between NdeI and BamHI sites of pHis17 to produce plasmid pDG64. A kanamycin resistance cassette, flanked by frt sites, was amplified from plasmid pKD4 (ref. 61 ) and cloned between the BamHI and HindIII restriction sites of pDG64 resulting in plasmid pDG65. For recombination, two of the following primers were used to PCR out the min operon encoding the msfGFP sandwich MinC fusion plus the kanamycin cassette from plasmid pDG65: forward primer: (dg173) ‘5′-GAA CAT CAT CGC GCG CTG GCG ATG ATT AAT AGC TAA TTG AGT AAG GCC AGG ATG TCA AAC ACG CCA ATC GAG CTT-3′’; reverse primer: (dg175) ‘5′-TCA AGG CAG AGA TAA CTC TGC CTT GAA GAT AAA TGC GCT TTT ACA GCG GGC TTA TGA ATA TCC TCC TTA GTT CCT-3′’. The forward primer (dg173) had 51 nt complementary sequence to the immediate upstream sequence of min operon followed by 24 nt complementary sequence to 5′-end of MinC. Similarly, the reverse primer (dg175) had 51 nt complementary sequence to the immediate downstream of min operon followed by 24 nt complementary sequence to the 3′-end of kanamycin cassette. The PCR product of dg173 and dg175 was gel purified and transformed into AB1157 cells overexpressing λ-Red proteins from pKD46 (ref. 61 ). After λ-Red integration, pKD46 plasmid was cured by growing the recombinant clones at 42 °C and finally selected for kanamycin resistance. The correct integration was assessed by PCR and sequencing. How to cite this article : Ghosal, D. et al. MinCD cell division proteins form alternating copolymeric cytomotive filaments. Nat. Commun. 5:5341 doi: 10.1038/ncomms6341 (2014). Accession codes: The coordinates for AaMinD and AaMinCD have been deposited in the Protein Data Bank under accession numbers 4V03 and 4V02 , respectively.